Super liquid-repellent gas membranes for carbon dioxide capture and heart–lung machines In a gas membrane, gas is transferred between a liquid and a gas through a microporous membrane. The main challenge is to achieve a high gas transfer while preventing wetting and clogging. With respect to the oxygenation of blood, haemocompatibility is also required. Here we coat macroporous meshes with a superamphiphobic—or liquid repellent—layer to meet this challenge. The superamphiphobic layer consists of a fractal-like network of fluorinated silicon oxide nanospheres; gas trapped between the nanospheres keeps the liquid from contacting the wall of the membrane. We demonstrate the capabilities of the membrane by capturing carbon dioxide gas into a basic aqueous solution and in addition use it to oxygenate blood. Usually, blood tends to clog membranes because of the abundance of blood cells, platelets, proteins and lipids. We show that human blood stored in a superamphiphobic well for 24 h can be poured off without leaving cells or adsorbed protein behind. In a gas contactor membrane, gas exchange is accomplished by passing the liquid and the gas on opposite sides of a microporous membrane [1] , [2] , [3] , [4] . By carefully controlling the pressure difference between the fluids, the liquid is immobilized in the pores of the membrane so that the interface is located at the mouth of each pore. Gas contactor membranes, in short gas membranes, are promising candidates for capturing carbon dioxide after its release, for example, in power plants or cement production, for sequestering or for use, for example, in methanol production [5] . Compared with conventional absorbers, gas membranes have a high active surface area, minimize flooding, foaming and entrainment, they have defined gas and liquid flow rates, are modular and easy to scale up [5] , [6] , [7] , [8] . In applications, gas membranes are, however, often plagued with problems such as wetting of the complete membrane (impalement), poor temperature stability, plugging and poor resistance to organic, acidic or basic solvents [5] . Synthetic nanoporous gas membranes are also used in biomedical applications including biosensing, biosorting, immunoisolation, drug delivery and the oxygenation of blood [9] , [10] . Conceptually, gas scrubbing and oxygenation of blood are similar. For the oxygenation of blood, clogging, haemolysis and platelet leakage are major problems [11] . A water or an oil drop placed on a superamphiphobic layer forms a contact angle greater than 150°. Tilting a superamphiphobic layer by a few degrees is already sufficient for a drop to overcome adhesion and to roll off. To achieve this liquid repellency, a superamphiphobic layer consists of microscopic protrusions having overhanging topography. The protrusions are fluorinated to render the surface hydrophobic [12] , [13] , [14] , [15] , [16] , [17] . A liquid drop placed on such a layer will trap air so that it physically separates the substrate from the liquid by a layer of gas. As the liquid rests on top of the protrusions, the real solid/liquid contact area is only a few percent of the apparent contact area [17] . Here, we demonstrate that superamphiphobic membranes can be used to exchange carbon dioxide. We further demonstrate that the human blood can be oxygenized by superamphiphobic membranes. Potential applications are extracorporal membrane oxygenators, for example, in heart–lung machines. Superamphiphobic membranes To achieve efficient gas exchange we coated membranes, in our case macroporous steel meshes, with a superamphiphobic layer ( Fig. 1a,b ). To make the layers a fractal-like layer of aggregated soot particles serves as a template for a highly porous silicon oxide layer [18] . After burning the soot away and coating the silicon oxide with perfluoroalkylsilane, an optically transparent, robust superamphiphobic layer is formed ( Fig. 1c–f , Supplementary Fig. S1 ). 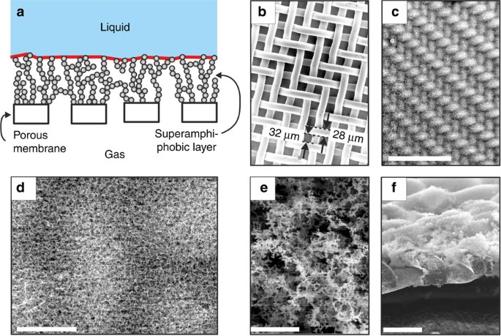Figure 1: Superamphiphobic membranes. (a) Schematic representation of a superamphiphobic gas membrane. The effective gas/liquid interface is highlighted in red. (b) SEM images of a stainless steel mesh (c–e) and after coating with an approximately 35 μm thick superamphiphobic layer. (f) Cross-section of the mesh showing that the wires are partially embedded in the layer. We did not observe an influence of the thickness of the coating on the gas exchange rate or on the anticlogging behaviour of the layer for thicknesses above 15 μm. Scale bars, 500 μm (c), 40 μm (d), 3 μm (e) and 60 μm (f). Figure 1: Superamphiphobic membranes. ( a ) Schematic representation of a superamphiphobic gas membrane. The effective gas/liquid interface is highlighted in red. ( b ) SEM images of a stainless steel mesh ( c – e ) and after coating with an approximately 35 μm thick superamphiphobic layer. ( f ) Cross-section of the mesh showing that the wires are partially embedded in the layer. We did not observe an influence of the thickness of the coating on the gas exchange rate or on the anticlogging behaviour of the layer for thicknesses above 15 μm. Scale bars, 500 μm ( c ), 40 μm ( d ), 3 μm ( e ) and 60 μm ( f ). Full size image To verify the superamphiphobicity of the meshes, we measured the contact angle Θ and the roll-off angle α for an aqueous solution of the surfactant SDS, peanut oil and n -hexadecane ( Table 1 ). In all cases, the contact angle is above 150° and the roll-off angle is below 10°. The superamphiphobic membrane is UV resistant, stable up to 400 °C ( Supplementary Fig. S2 ), and does not swell in organic or polar liquids. It is highly porous with approximately 90–95 vol% gaseous phase ( Supplementary Fig. S3 ). Table 1 Contact angle and roll-off angle for liquid of 6±1 μ l volume on a superamphiphobic mesh. Full size table Uptake of carbon dioxide To measure carbon dioxide uptake, the pH indicator phenolphthalein (pK a =9.7) was added to an aqueous solution of 0.22 M NaOH (pH 13). As long as the solution was kept in a nitrogen atmosphere, the typical pink colour of deprotonated phenolphthalein was observed, resulting from an absorption peak at 555 nm ( Supplementary Fig. S4 ). When introducing carbon dioxide into the gas box the absorption first increased ( Fig. 2b,c ). The increase is caused by shift of the pH from 13 to 11.5, where the absorption is maximal. [19] Then the absorption decreased to zero, reflecting a reduction in pH to below 8.2. Carbon dioxide diffused into the aqueous solution, and reacted with water to form carbonic acid, which neutralized the NaOH (CO 2 +2NaOH→Na 2 CO 3 +H 2 O). This carbon dioxide capture verifies that superamphiphobically coated meshes can indeed be used as gas contactor membranes. From the changing absorption, we estimated the mass transfer coefficient K . The transfer coefficient is the amount of gas crossing the membrane per unit time and area divided by the driving concentration difference. As a lower limit, we find K =5.3 × 10 −4 m s −1 for the exchange of carbon dioxide. This value is comparable to highly efficient gas contactor membranes [20] , [21] . A potential advantage of superamphiphobic gas membranes is that, in addition to aqueous solutions, other absorbing liquids can be used such as aqueous amine solutions or ionic liquids [22] , [23] , [24] . The technique also holds promise to scrub other gases, for example, H 2 S or silanes. 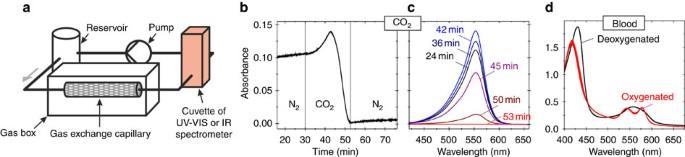Figure 2: Gas exchange. (a) Sketch of the set-up used to measure gas exchange. Gas was exchanged in the gas box through a superamphiphobic tube or a flow cell. (b) Neutralization of basic aqueous solution. Absorbance at 555 nm of an aqueous solution with 0.22 M NaOH and 0.18 mM phenolphthalein. The total volume of the entire system was 18 ml. Att=30 min, the nitrogen atmosphere was exchanged for carbon dioxide. A superamphiphobically coated elliptical flow cell was used. (c) Full UV–VIS spectra of the solution at different stages of neutralization. (d) Absorbance spectra of 1.2% deoxygenated blood before and after exposure to oxygen. When exposing deoxygenated blood to O2via a superamphiphobic porous tube, the absorption spectrum developed the characteristic double peak at 560 nm within 9 min. The UV-VIS spectrum of haemoglobin is dominated by its metal–ligand interaction. The electronical structure of the metal-ligand systems changes because of the oxygenation of deoxyhaemoglobin to oxyhaemoglobin, causing the changes of the UV-VIS spectra. Figure 2: Gas exchange. ( a ) Sketch of the set-up used to measure gas exchange. Gas was exchanged in the gas box through a superamphiphobic tube or a flow cell. ( b ) Neutralization of basic aqueous solution. Absorbance at 555 nm of an aqueous solution with 0.22 M NaOH and 0.18 mM phenolphthalein. The total volume of the entire system was 18 ml. At t =30 min, the nitrogen atmosphere was exchanged for carbon dioxide. A superamphiphobically coated elliptical flow cell was used. ( c ) Full UV–VIS spectra of the solution at different stages of neutralization. ( d ) Absorbance spectra of 1.2% deoxygenated blood before and after exposure to oxygen. When exposing deoxygenated blood to O 2 via a superamphiphobic porous tube, the absorption spectrum developed the characteristic double peak at 560 nm within 9 min. The UV-VIS spectrum of haemoglobin is dominated by its metal–ligand interaction. The electronical structure of the metal-ligand systems changes because of the oxygenation of deoxyhaemoglobin to oxyhaemoglobin, causing the changes of the UV-VIS spectra. Full size image A major factor that limits the performance of gas contactor membranes is wetting. Organic and biological liquids tend to spread on flat hydrophobic surfaces, even on teflon, implying wetting of the pores of membranes. The reason is that the completely wetted state is energetically more favourable than the desired state where air is trapped. However, the geometry of superamphiphobic surfaces creates an energy barrier that prevents liquid from penetrating in the pores. This holds until a certain critical pressure, the impalement pressure, is exceeded. For superamphiphobic membranes consisting of nanospheres this pressure can be estimated to be [17] here γ is the surface tension of the liquid, R is the radius of the nanospheres, r is the minimal distance between protrusions and Θ m is the advancing material’s contact angle of the liquid on a flat fluorinated surface. In our case and for a 21 w% aqueous amine solution with γ =0.053 N m −1 , with R =50 nm, r =1 μm and Θ m =120° the theoretical impalement pressure is P c =4 kPa. Practically, with our not-yet-optimized design, we could support a 30 cm aqueous amine column (3 kPa). Large air domains between adjacent wires should be avoided because they reduce the impalement pressure ( Supplementary Fig. S1 ). Oxygenation of blood To demonstrate oxygenation of blood, we first deoxygenized a 1.2% solution of whole human blood stabilized with lithium-heparin as an anticoagulant in PBS (Dulbecco’s PBS) by bubbling a continuous stream of nitrogen through the solution for 30 min at 37 °C; blood was diluted to reach a high sensitivity in the UV/VIS absorption spectrometer. Deoxygenated blood in PBS was transferred into the reservoir of the set-up ( Fig. 2a ) under nitrogen. We continuously recorded UV/VIS absorption spectra. Diluted blood circulated for 16 min under nitrogen atmosphere until oxygen was introduced into the gas box at a flow rate of 0.7 l min −1 . Spectra measured at t =0 min and t =45 min demonstrate that pumped blood in PBS was successfully oxygenated ( Fig. 2d ). The solution was pumped for more than 1 h in a closed system without any leakage of diluted blood. Interaction of blood with superamphiphobic layers When we opened the elliptical flow cell after perfusion with diluted or whole human blood solution, no blood was left behind on the superamphiphobic coating, proving its blood repellency ( Fig. 3b ). In contrast, a piece of Teflon left in the flow cell was covered with blood ( Fig. 3a ). SEM images of a flow cell taken after whole human blood was circulating for 3 h were almost undistinguishable from those taken before the start of the measurement ( Supplementary Fig. S5 ). 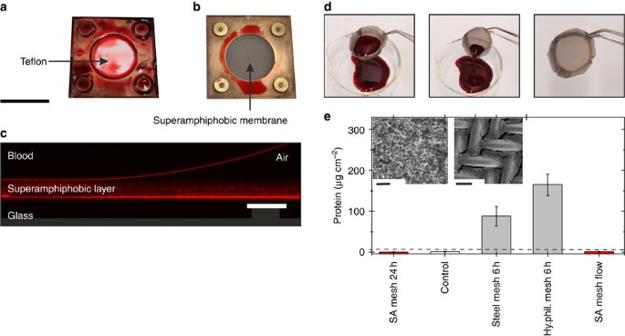Figure 3: Adsorption of blood on superamphiphobic membranes. Whole human blood was pumped through a flow cell equipped with two teflon layers (a) or with two superamphiphobic meshes (b). Afterwards the cells were opened and the pictures were taken. (c) Vertical cross-section of a drop of blood on a superamphiphobic layer imaged with a confocal microscope in a reflection mode (supporting information). Reflected light from the superamphiphobic layer, from the blood-air and from the glass-air interface shows that blood does not wet the membrane. (d) Whole human blood rinsed out of a superamphiphobically coated basket made of a steel mesh (Supplementary Movie 1). (e) Results of the protein adsorption assay. The amount of protein adsorbed was measured for (from left to right) the following: a superamphiphobically coated steel mesh after 24 h exposure to non-flowing blood; a control superamphiphobic mesh, which had never been in contact with blood; a bare, uncoated steel mesh after exposing it to non-flowing blood for 6 h; a coated but unfluorinated steel mesh after 6 h exposure to non-flowing blood (Hy.phil. mesh). In addition, a superamphiphobic steel mesh was exposed to a blood flow (5.12 ml min−1) for 3 h. Washing of the samples (three times with 3 ml PBS) removed blood that did not adhere to the surface. Error bars are based upon the root mean square deviation. The horizontal dashed line is the detection limit of 6 μg cm−2. Inset: (left) SEM image of a superamphiphobic membrane after 48 h exposure to whole human blood; (right) SEM image of the corresponding metal mesh after 2 h exposure to whole human blood. Scale bars, 2 mm (a,b), 50 μm (c), 10 μm (e, left) and 50 μm (e, right). Figure 3: Adsorption of blood on superamphiphobic membranes. Whole human blood was pumped through a flow cell equipped with two teflon layers ( a ) or with two superamphiphobic meshes ( b ). Afterwards the cells were opened and the pictures were taken. ( c ) Vertical cross-section of a drop of blood on a superamphiphobic layer imaged with a confocal microscope in a reflection mode (supporting information). Reflected light from the superamphiphobic layer, from the blood-air and from the glass-air interface shows that blood does not wet the membrane. ( d ) Whole human blood rinsed out of a superamphiphobically coated basket made of a steel mesh ( Supplementary Movie 1 ). ( e ) Results of the protein adsorption assay. The amount of protein adsorbed was measured for (from left to right) the following: a superamphiphobically coated steel mesh after 24 h exposure to non-flowing blood; a control superamphiphobic mesh, which had never been in contact with blood; a bare, uncoated steel mesh after exposing it to non-flowing blood for 6 h; a coated but unfluorinated steel mesh after 6 h exposure to non-flowing blood (Hy.phil. mesh). In addition, a superamphiphobic steel mesh was exposed to a blood flow (5.12 ml min −1 ) for 3 h. Washing of the samples (three times with 3 ml PBS) removed blood that did not adhere to the surface. Error bars are based upon the root mean square deviation. The horizontal dashed line is the detection limit of 6 μg cm −2 . Inset: (left) SEM image of a superamphiphobic membrane after 48 h exposure to whole human blood; (right) SEM image of the corresponding metal mesh after 2 h exposure to whole human blood. Scale bars, 2 mm ( a , b ), 50 μm ( c ), 10 μm ( e , left) and 50 μm ( e , right). Full size image For the oxygenation of blood and for all long-term applications, an additional demand is that attachment of blood cells and clogging must be suppressed. To test the wetting and anticlogging properties, a drop of fresh human blood was placed on a horizontal, planar superamphiphobic mesh. It formed an advancing contact angle of Θ=162±1° and rolled off when tilting the mesh by α =5±1°. Superamphiphobic layers were not impaled by blood as verified by confocal microscopy on superamphiphobically coated glass ( Fig. 3c ). In contrast, blood impales superhydrophobic surfaces because blood has a low surface tension of γ =47 mN m −1 ( Supplementary Fig. S6 ). Furthermore, we shaped superamphiphobically coated meshes into small wells or baskets, filled them with full human blood and incubated them up to 48 h at 37 °C in saturated atmosphere; resting liquid facilitates attachment as compared with a flowing liquid. Remarkably, the blood rolled off without leaving any visible traces ( Fig. 3d , Supplementary Movie 1 ). No blood cells could be found by optical or scanning electron microscopy (SEM) even after 48 h incubation ( Fig. 3e , Supplementary Fig. S7 ). Contrary, blood wets the metal meshes causing strong adhesion of blood on the meshes ( Fig. 3e , Supplementary Fig. S8 ). Such a low adhesion from pure solid surfaces has, to our knowledge, not been observed yet. The only directly comparable experiments we know of were carried out with slippery fluorinated liquid-infused porous surfaces [25] . The fluorinated molecules are not linked to the surface but applied as a liquid. Blood could be rinsed off after few minutes of exposure. The release of fluorinated molecules could, however, not be excluded. In the present approach, the fluorosilanes are covalently linked to the silicon oxide, greatly reducing the likeliness that fluorinated molecules can be released. We also measured the adhesion of proteins from human blood, as proteins adsorb to all types of surfaces, both charged and uncharged. The amount of adsorbed proteins is a measure of haemocompatibility, and adsorption is usually the first step in biofilm formation [26] , [27] , [28] , which must be prevented. We compared superamphiphobically coated meshes with bare steel meshes and with meshes coated with a layer of soot-templated silicon oxide without fluorination ( Fig. 3e ). When exposing the superamphiphobic layer to stationary blood even for 24 h, no adsorption was detected. In contrast, on the bare steel mesh and the hydrophilic mesh after 6 h we observed significant protein adsorption. This hints towards good haemocompatibility, likely caused by the greatly reduced contact area between blood with the artificial surface. Efficient, nonwetting, antiplugging gas exchange membranes could be fabricated by coating macroporous membranes with a superamphiphobic layer. These newly designed superamphiphobic membranes may also advance chemical processing, for example, enable more efficient gases scrubbing even with non-aqueous liquids, and food processing, for example, in the beverage industry. The efficient gas transfer may allow a reduction in the volume of scrubbing solvent. The combination of efficient gas exchange and low attachment of blood cells (anticlogging, no platelet leakage, good haemocompatibility) holds promise for biomedical applications, for example, as blood oxygenators. The antiwetting property of superamphiphobic layers makes them attractive as coating for vessels and tubes used to store and transport blood. Superamphiphobic membranes Stainless steel meshes with a width of 32 μm ( Fig. 1b ) were cleaned by supersonicating in water, ethanol and water for 15 min, respectively. After drying in air, soot from paraffin candles was collected 1.5–1.8 cm above the wick. Collection times of soot depended on the size of the substrate and the desired layer thickness. A 10–40 μm-thick layer of soot was deposited. The soot consists of carbon particles with diameters of 30–50 nm, forming a loose, fractal-like network [29] . The sooting time determined whether the porous superamphiphobic mesh was coated with a homogeneous layer or whether the wires were well-separated by μm-sized air domains ( Supplementary Fig. S9 ). This template of soot particles was coated with a 30–40 nm thick layer of porous silicon oxide ( Fig. 1c–f ) by chemical vapour deposition(CVD) of tetraethylorthosilicate (TEOS). Therefore, soot-coated meshes were transferred to a desiccator. Two open glass vessels (diameter 2 cm, volume 30 ml) were placed next to the samples. One was filled with 3 ml aqueous ammonium hydroxide solution 28% (Normapur), the other one was filled with 3 ml TEOS. The desiccator was sealed and the pressure was reduced to 250 m bar. After 1 min, the desiccator valve was slightly opened to slowly release the vacuum. CVD of TEOS lasted 24 h. Then the soot was burned away at 600 °C for 3 h in an oven in air. To hydrophobize the meshes after combustion they were placed into a desiccator. A glass vessel, filled with 300 μl trichloro(1H,1H,2H,2H-perfluorooctyl)silane, was placed next to the meshes. The pressure in the desiccator was reduced to 250 mbar, and the meshes were allowed to silanize for 2 h. Gas exchange Gas was exchanged in an elliptical flow cell (transverse diameter 2 cm, conjugate diameter 0.8 cm) with 3 mm spacing between two parallel superamphiphobically coated meshes, resulting in an entire volume of 0.38 cm 3 and an active filter area of 2 × 1.25 cm 2 ( Supplementary Fig. S10 ). Alternatively, we used superamphiphobically coated capillaries for gas exchange. Therefore, superamphiphobically coated meshes were shaped into tubes by hand with the nanoporous layer pointing inward (inner diameter: 2.5–3 mm, length: 3–6 cm). Therefore, steel meshes of 3 to 6 × 1 cm 2 were covered on one or both sides with an approximately 30 μm thick layer of soot. Afterwards the soot template was stabilized by chemical vapour deposition of TEOS for 24 h. The coated meshes were combusted at 600 °C for 2 h. After calcination the meshes were shaped into capillaries by hand with the layer pointing inward (inner diameter: 2.5–3 mm, length: 3–6 cm). The inner surface area was 2.4–5.7 cm 2 . The shape was permanently fixed by wrapping a (copper) wire around them. Finally, capillaries were hydrophobized by CVD of trichloro(1H,1H,2H,2H-perfluorooctyl)silane for 2 h. The capillaries were fixed by heat-shrink tubing to stainless steel tubes of the set-up. The flow cell or tube was connected to a tubing pump (5.1 ml min −1 ), a reservoir and a UV-VIS flow cuvette ( Fig. 2a ). The cell was placed into a gas tight box, which was equipped with two valves for in- and out-flowing gas (see supporting information for a detailed description). Thermal stability To quantify the thermal stability, a superamphiphobic layer was annealed at temperatures of 100, 200, 300, 400 and 450 °C for 1 h ( Supplementary Fig. S2 ). The static contact and roll-off angles remained constant up to 400 °C. Annealing at even higher temperatures decomposed the fluorosilane. Furthermore, the temperature resistance of the coating depends on time. The maximum temperature until the coating loses its liquid repellency decreases with annealing duration. The silica network remained almost unaltered until annealing up to 1,000 °C [18] . CO 2 /NaOH-neutralization as function of wavelength Spectra were recorded from 350 to 700 nm every 80 s. The spectra showed the typical UV/VIS absorbance of basic phenolphthalein solution (absorption maximum at 555 nm). After 30 min, the gas tight box was flushed with CO 2. The absorbance at 555 nm dropped from a former constant value of 0.14 to a constant background value of ca. 0.01. For lower NaOH concentrations the neutralisation proceeds in less than one flow cycle what corresponds to less than 80 s ( Supplementary Fig. S4 , left). In this case, the neutralization of the through flowing sodium hydroxide solution can also easily be confirmed by eye ( Supplementary Fig. S4 , right): Before flushing the chamber with CO 2 , in- and outflow were clearly pink. After CO 2 flush, the inflow (coming from the reservoir) was still pink and the outflow was transparent as the inflowing sodium hydroxide solution was neutralized by CO 2 diffusing through the membrane placed in the chamber. Estimation of the mass transfer coefficient for CO 2 From the changing absorption, we can estimate the mass transfer coefficient K of CO 2 . The mass transfer coefficient is defined as the amount of gas transferred per time and per unit area A divided by the driving concentration difference . The driving concentration difference is Δ c = P/k H − c l . Here k H =29.4 atm M −1 is Henry’s constant for CO 2 and water at 25 °C, and c l is the mean concentration of CO 2 in water. P/k H is the concentration of CO 2 in water equilibrated with CO 2 gas at pressure P . We further assume that the concentration of CO 2 in the liquid is negligible ( c l =0), as it will be consumed by the neutralization reaction. This is a rough assumption because the conversion rate of CO 2 to H 2 CO 3 in water is known to be slow (0.039 s −1 ). Therefore, we calculate a lower limit for the mass transfer coefficient. We take the increase in absorption to estimate the transfer coefficient (minimum 35–42 in Fig. 2b ). In this range from pH 13 to 11.5 most of the NaOH is neutralized. The total amount of NaOH neutralized in 7 min is 3.8 × 10 −3 mol (0.22 M times the total liquid volume of 17.5 ml). As the reaction is carried out above the second pK of carbonic acid of 10.3, every carbon dioxide neutralizes two NaOH molecules (H 2 CO 3 +2 NaOH→Na 2 CO 3 +2H 2 O). This leads to a transfer rate =4.5 × 10 −6 mol s −1 . With an apparent membrane area of 2.5 × 10 −4 m 2 and P =1 atm we obtain a mass transfer coefficient K =5.3 × 10 −4 m s −1 . This value is a lower limit because we assumed that CO 2 is immediately converted to carbonic acid and because we used the mean decreases in hydroxyl concentration in the 7 min considered rather than the maximal decreases. This is already of the same order of magnitude as highly efficient conventional gas contactor membranes [20] , [21] . Laser scanning confocal microscopy of blood Superamphiphobic layers are transparent because of their high air fraction of larger than 90%. To verify that blood does not wet these layers, confocal microscopy pictures were taken with an inverted Leica TCS SP5 II—STED CW confocal microscope. Drops of whole or diluted blood were deposited on a glass slide coated with a superamphiphobic layer, prepared in the same way as the superamphiphobically coated meshes. All measurements were carried out in reflection mode, and thus no labelling was required. A dry objective with high numerical aperture ( × 40/0.85) allowed for high axial resolution of 1.0 μm and measurement of reflected light even from tilted surfaces. The large differences between the refractive indices of blood (~1.33), air (1.0), glass and silica (~1.5) gave rise to strong reflections from all interfaces. The superamphiphobic layer consists mostly of air, and thus its refractive index is close to 1. Thus, the horizontal glass-superamphiphobic layer and the blood-superamphiphobic layer interfaces were clearly visible in Fig. 3c . The blood-air interface was curved because of the small size of the drop (about 2 mm in diameter). The superamphiphobic layer itself was visible as a diffuse pattern, resulting from the silica nanoparticles. Even after 1 h, no change in the height of the blood-superamphiphobic layer was observed, verifying that blood does not wet this layer. Adhesion of resting blood on a metal mesh Blood was deposited on a metal mesh without any further movement for 2 h ( Supplementary Fig. S8 ). Blood wetted the mesh immediately. After the blood was removed the mesh was investigated by scanning electron microscopy. A mixture of proteins and blood cells entirely covered the metal mesh. The size of blood cells greatly exceeds the average distance between neighbouring protrusions of the superamphiphobic coating. The substructure of the superamphiphobic coating (SiO 2 particles in the range of 40 nm) is even two orders of magnitude smaller than the 8-μm-sized red blood cells. Measurement of protein adsorption First, steel meshes were shaped into wells ( Fig. 3d ). Three different kinds of meshes were investigated: superamphiphobic, hydrophilic and untreated metal mesh wells. Superamphiphobic wells were obtained by coating metal meshes by the method mentioned before [18] . Hydrophilic meshes were fabricated in analogy to the superamphiphobically coated meshes. Only the last step, the hydrophobization of the soot-templated silicon oxide was not carried out. Two wells of each kind were placed in a six-well plate. 2 ml of whole human blood were filled into each well. The samples were covered with a moist filter paper, and the lid was sealed with Parafilm to reduce evaporation. The six-well plates were transferred to an incubator at 37 °C for 6 or 24 h at rest. After the specified time, the blood was removed by tilting the wells ( Fig. 3d ). Then the wells were washed three times with 1 ml PBS. Only the surface area of the wells that were in direct contact with the supernatant blood was analysed quantitatively. Therefore the investigated mesh parts were cut into small pieces. These pieces were incubated in 5% SDS and 2.3% dithiothreitol (DTT) for 5 min at 95 °C with constant agitation to desorb all proteins. To remove possible particulate contamination from the mesh, the solutions were centrifuged for 10 min at 15,000 g . The amount of protein in the supernatant was measured using the Pierce 660 nm Protein Assay Kit. Thereby, proteins were fluorescently labelled, and the total amount of protein in a sample was identified by measuring the fluorescence of the sample and comparing it with a calibration curve. Each sample was measured in triplicates. Protein concentrations were determined using reagent supplemented with Ionic Detergent Compatibility Reagent (Thermo Scientific; Germany) according to manufacturer’s instructions with BSA as a standard. In parallel, the mesh pieces were weighed to calculate the surface area. The amount of protein was divided by the calculated surface area of the mesh for every sample. Scalability The size of the superamphiphobic meshes were limited by size of processing equipment (oven, desiccators). Soot collection could further be scaled up by specific industrial sooting devices (for example, Evonic is running such devices to produce defined soot for car tires). How to cite this article: Paven, M. et al. Super liquid-repellent gas membranes for carbon dioxide capture and heart–lung machines. Nat. Commun. 4:2512 doi: 10.1038/ncomms3512 (2013).